Histone demethylase KDM5A is regulated by its reader domain through a positive-feedback mechanism The retinoblastoma binding protein KDM5A removes methyl marks from lysine 4 of histone H3 (H3K4). Misregulation of KDM5A contributes to the pathogenesis of lung and gastric cancers. In addition to its catalytic jumonji C domain, KDM5A contains three PHD reader domains, commonly recognized as chromatin recruitment modules. It is unknown whether any of these domains in KDM5A have functions beyond recruitment and whether they regulate the catalytic activity of the demethylase. Here using biochemical and nuclear magnetic resonance (NMR)-based structural studies, we show that the PHD1 preferentially recognizes unmethylated H3K4 histone tail, product of KDM5A-mediated demethylation of tri-methylated H3K4 (H3K4me3). Binding of unmodified H3 peptide to the PHD1 stimulates catalytic domain-mediated removal of methyl marks from H3K4me3 peptide and nucleosome substrates. This positive-feedback mechanism—enabled by the functional coupling between a reader and a catalytic domain in KDM5A—suggests a model for the spread of demethylation on chromatin. The dynamic interplay of post-translational modifications (PTMs) on histone tails in nucleosomes provides a molecular mechanism for responding to cellular stimuli by regulating chromatin structure and function [1] , [2] . Among the numerous PTMs on histone tails, histone lysine methylation plays a crucial role in controlling gene expression [1] . The dynamics of lysine methylation on chromatin is tightly regulated by the coordinated function of enzymes and proteins that ‘write’, ‘read’ and ‘erase’ this mark [3] . Removal of lysine methyl marks from chromatin is carried out by histone demethylases. Flavin-dependent demethylases LSD1 and LSD2 act on a subset of mono- and di-methylated lysine residues, and the broader and more recently discovered jumonji C (JmjC) domain-containing demethylase family acts on a wide range of mono-, di- and tri-methylated lysine substrates. Contrary to histone lysine methyltransferases (KMTs), where extensive in vitro and in vivo studies have been conducted to characterize their activity on chromatin, there is limited information on the mechanisms that control the activities of histone lysine demethylases (KDMs), and in particular the jumonji family. Yet, the need to mechanistically dissect the function of histone KDMs on chromatin rests on the mounting evidence that JmjC domain-containing KDMs are important during development and are misregulated in several cancers and neurological disorders [4] , [5] , [6] , [7] , [8] . KDM5A (RBP2, JARID1A) belongs to the KDM5 subfamily of Jumonji histone demethylases that act on tri-, di- and mono-methylated lysine 4 of histone H3 (H3K4me3/2/1). The KDM5 family also includes PLU-1/KDM5B, SMCX/KDM5C and SMCY/KDM5D. The KDM5 enzymes share a highly conserved domain architecture that includes a JmjN domain, the catalytic JmjC domain, a Bright/Arid DNA binding domain, a C 5 HC 2 zinc finger and two or three PHD domains. Originally described as a binding partner of the tumour suppressor retinoblastoma protein, KDM5A is a critical transcriptional regulator in cellular differentiation and development [9] , [10] , [11] , [12] , [13] , [14] . KDM5A overexpression promotes tumorigenesis and drug tolerance in cancer cells and thus represents a potential therapeutic target [6] , [15] , [16] , [17] , [18] . Despite its importance in physiology and disease, the mechanisms by which the demethylase activity of KDM5A, and KDM5 demethylases in general, are regulated on chromatin are unknown. Plant homeodomain (PHD) fingers contain a Cys 4 HisCys 3 motif that coordinates two zinc ions in a cross-brace manner and have emerged as sequence- and modification-specific histone recognition domains [19] , [20] , [21] , [22] , [23] . To date, PHD domains in demethylases and demethylation complexes have been shown to act as binding modules to regulate occupancy and substrate specificity of demethylases [24] , [25] , [26] , [27] . To investigate whether the functions of PHD domains in demethylases extend beyond recruitment and could contribute to the regulation of the catalytic activity of these enzymes, we set out to interrogate their roles in the context of KDM5A. Among the three PHD domains of KDM5A, PHD3 has been studied in the context of its fusion with nucleoporin NUP98 where it has been shown to specifically bind to the H3K4 tri-methyl mark [28] . While the function of the PHD2 domain is not known; qualitative pull-down assays with isolated PHD1 domain of KDM5A suggest that this domain binds unmodified H3K4 peptide [28] . Yet, the functional relevance of this binding and its potential impact on the demethylation activity of KDM5A is unknown. Clues to a regulatory role follow from experiments showing that deletion of PHD1, but not PHD2 or PHD3, in human and Drosophila KDM5A homologues abrogates their enzymatic activity in vivo , increasing cellular H3K4me3 levels [29] , [30] . Furthermore, in the primary sequence of the demethylase, the PHD1 is positioned between the JmjN and JmjC domains, which have been postulated to form a composite active site in KDM5 histone demethylases [29] , [31] , [32] . These observations suggest a potential role of the PHD1 domain in regulating the catalytic activity of KDM5A. The PHD1 preferentially recognizes H3K4me0 histone tails To interrogate the function of the PHD1 domain and obtain a quantitative estimate of its histone tail-binding specificity, we first cloned and recombinantly expressed a glutathione S-transferase (GST) fused PHD1 291–347 construct. Using a fluorescence polarization (FP)-based assay, we monitored its association with fluorescently labelled histone H3, H4, H2A and H2B tail peptides ( Fig. 1b ). Of all four histone tail peptides, the PHD1 domain recognized only the histone H3 tail with low micromolar affinity, a strength of interaction comparable to other histone binding PHD domains ( Fig. 1b,d ). The binding of the PHD1 domain to the H3 tail peptide was lost when the first four residues, ARTK, were removed (H3 5–18 ) ( Fig. 1b ). Moreover, using unmethylated and methylated H3 tail peptides, we found that the PHD1 domain prefers the H3 peptide that contains unmethylated Lys4 (H3K4me0), and shows the lowest affinity for the H3 tail peptide in which Lys4 is tri-methylated (H3K4me3; Fig. 1c,d ). While Lys4 methylation provides a selectivity filter, the presence of the lysine side chain is not required for binding ( K d of the mutant peptide in which Lys4 is mutated to an Ala (K4A peptide) is 2 μM, Fig. 1d ). In contrast, mutation of the arginine at position 2 (R2) to alanine results in more than 25-fold decrease in affinity ( K d R2A peptide=49 μM, Fig. 1d ). Dimethylation of R2, either symmetric (H3R2me2s) or asymmetric (H3R2me2a), reduces binding affinity by approximately fivefold ( Fig. 1d ). While methylation of both R2 and K4 influences peptide binding to the PHD1, methylation of lysine 9 has no effect on PHD1 binding ( Supplementary Fig. 1 ). Together, these results suggest that the PHD1–H3 tail interaction is sensitive to the methylation status of both R2 and K4 residues. The preference for unmethylated H3 tail peptides parallels the specificity of the PHD1 domain of Drosophila homologue Lid [30] and the PHD1 domain in KDM5B (refs 33 , 34 ). These findings suggests that the preferential binding of unmodified lysine 4 in histone H3 may be an evolutionarily conserved feature of this reader domain in the KDM5 family of demethylases. 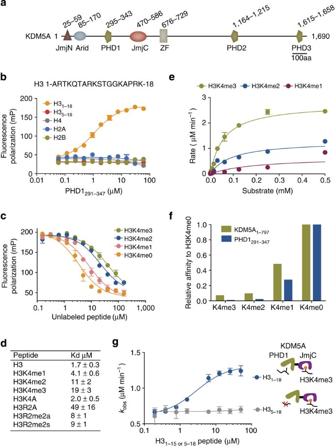Figure 1: KDM5A PHD1 recognizes the N-terminal region of the H3 tail and this binding stimulates H3K4me3 demethylation by KDM5A. (a) KDM5A domain map. (b,c) Binding of peptides to PHD1 assessed by fluorescence polarization: (b) histone tail peptides (amino acids 1–18 and H3 5–18); (c) peptides with different degrees of methylation on lysine 4 of histone H3. (d) Dissociation constants for different histone H3 peptides (1–18 aa). (e) Demethylation activity of KDM5A1–797towards methylated H3K4 histone tail peptides. (f) Affinity measurements, relative to the H3K4me0 peptide, of KDM5A PHD1 and KDM5A1–797to H3 tail peptides with different extent of methylation on K4. (g) Stimulation of H3K4me3 demethylation by WT KDM5A1–797demethylase with increasing concentration of H31–18and H35–18effector tail peptides. Errors (n≥3) represent s.e.m. Figure 1: KDM5A PHD1 recognizes the N-terminal region of the H3 tail and this binding stimulates H3K4me3 demethylation by KDM5A. ( a ) KDM5A domain map. ( b , c ) Binding of peptides to PHD1 assessed by fluorescence polarization: ( b ) histone tail peptides (amino acids 1–18 and H3 5–18); ( c ) peptides with different degrees of methylation on lysine 4 of histone H3. ( d ) Dissociation constants for different histone H3 peptides (1–18 aa). ( e ) Demethylation activity of KDM5A 1–797 towards methylated H3K4 histone tail peptides. ( f ) Affinity measurements, relative to the H3K4me0 peptide, of KDM5A PHD1 and KDM5A 1–797 to H3 tail peptides with different extent of methylation on K4. ( g ) Stimulation of H3K4me3 demethylation by WT KDM5A 1–797 demethylase with increasing concentration of H3 1–18 and H3 5–18 effector tail peptides. Errors ( n ≥3) represent s.e.m. Full size image PHD1 occupancy stimulates peptide demethylation Our data indicate that the PHD1 domain in KDM5A preferentially recognizes H3 tail peptides that are unmethylated and, to a lesser extent, mono-methylated at K4 over those containing higher methylation states of this residue ( Fig. 1c,d ). As these preferred binding substrates are the products of KDM5A-mediated demethylation, this observation raises the possibility that the demethylation activity of this enzyme is regulated by a positive-feedback mechanism. To investigate this possibility and to isolate the role of PHD1 from PHD2 and PHD3, we used a KDM5A construct lacking the PHD2 and PHD3 domains ( Fig. 1a , KDM5A 1–797 ). We first evaluated the catalytic activity of this construct on H3K4me3, 2 and 1 methylated peptides using an enzyme-coupled fluorescent assay [35] . We found that KDM5A 1–797 demethylates all the H3K4 methylation states, with a preference for the H3K4 tri-methylated substrate ( Fig. 1e and Supplementary Table 1 ), consistent with previous findings [13] . Compared with previous in vitro studies on KDM5A (refs 13 , 14 ), however, we also detected demethylation of H3K4me1 peptides ( Supplementary Fig. 2 ). While this discrepancy could be due to differences in experimental conditions, our results are consistent with the observation that in vivo KDM5A can demethylate all three methylation states of K4. We then evaluated the binding selectivity of KDM5A 1–797 towards differentially methylated H3K4 peptides. In analogy to the isolated PHD1, KDM5A 1–797 preferentially binds unmethylated and mono-methylated H3K4 peptides compared with di- and tri-methylated H3K4 peptides ( Fig. 1f ), suggesting that the function of the PHD1 is retained in the context of the demethylase. To test whether binding of the ligand peptide to the PHD1 domain impacts the demethylase activity of KDM5, we compared the activity of the KDM5A 1–797 construct towards a H3K4me3 peptide in the presence of unmodified H3 1–18 peptide, ligand for the PHD1 or a truncated H3 5–18 peptide that does not bind to the PHD1 ( Fig. 1b,g ). Interestingly, we found that the demethylase activity was stimulated in the presence of H3 1–18 peptide, but no stimulation was observed with the control H3 5–18 peptide ( Fig. 1g ). We also observed a decrease in the catalytic rate of the enzyme at high H3 1–18 peptide concentrations (>50 μM) and attributed such effect to inhibition of the active site by this peptide. These results suggest a model whereby binding of an effector peptide to the PHD1 domain allosterically stimulates the activity of the catalytic domain. NMR structural analysis of the H3 tail-binding site in PHD1 To gain insight into the mode of recognition of H3 tail peptide by PHD1 and to identify residues that, when mutated, disrupt the PHD1–H3K4 tail complex, we employed nuclear magnetic resonance (NMR). The two-dimensional heteronuclear single quantum coherence (2D 15 N-HSQC) spectrum of the apo PHD1 revealed a well-dispersed set of cross-peaks that were assigned to residues by triple-resonance backbone experiments ( Fig. 2a ). The measured chemical shifts ( 1 H n , 15 N, 1 Hα, 13 Cα and 13 Cβ) were used to generate a CS-Rosetta model of the apo PHD1 domain ( Fig. 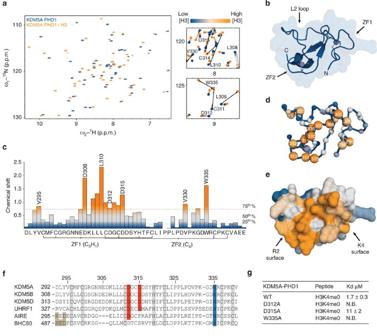Figure 2: Structure and H3 binding properties of KDM5A PHD1. (a) Backbone regions of the HSQC spectra of the apo and H3-bound forms of KDM5A PHD1. The apo and H3-bound spectra are coloured blue and orange, respectively. Insets show titration across key structural regions. (b) CS-Rosetta model of the apo KDM5A PHD1, consistent with the lowest energy and dihedral restraint considerations. (c) Normalized change in chemical shift (Hn, N, Hα, Cα and Cβ) by residue on H3 binding. Dashed lines indicate 25th, 50th and 75th percentile rankings, and colour gradient is such that unperturbed (<25th percentile) positions are in blue and significantly perturbed (>75th percentile) are in orange. (d) CS-Rosetta model of KDM5A PHD1 with backbone amides drawn as spheres, coloured by chemical shift perturbation. Selected residue numbers are indicated. (e) Surface representation of the KDM5A PHD1 coloured by chemical shift perturbations reveals the H3 binding surface. (f) Sequence alignment of KDM5A PHD1 to close homologues. Zinc coordinating residues are highlighted in grey, the conserved tryptophan in blue and aspartate residues proposed to coordinate H3R2 are highlighted in red. The residues that interact with H3K4 are highlighted in light brown. (g) Effect of mutations on KDM5A PHD1 recognition of unmodified H3 peptide (NB=no binding,KD>100 μM. Errors (n≥3) represent s.e.m.). 2b and Supplementary Figs 3 and 4 ) that was filtered by agreement with measured dihedral restraints ( Supplementary Table 2 ). While very similar to the structures of canonical PHD finger domains and, in particular, to the recently determined NMR structure of the PHD1 of KDM5B (ref. 34 ), the CS-Rosetta models reveal a novel ‘open’ conformation of the L2 loop (residues 323–335; Fig. 2b and Supplementary Fig. 5 ). On titration with the H3K4me0 peptide, we observed large changes in chemical shifts for many cross-peaks in the PHD1 spectra, consistent with direct binding ( Fig. 2a,c and Supplementary Fig. 6 ). Chemical shift changes were mapped onto the model of the apo PHD1 to display an extended peptide binding site ( Fig. 2d,e ). The largest perturbations were observed for the residues leading into the first β-strand (Glu305-Asp306), the first β-strand itself (β1, Leu308-Leu310) and the region that harbours the second Zn finger (Cys311-Asp315; Fig. 2c–e ). Large chemical shift perturbations were also detected close to the C terminus of PHD1 (Val330-Trp335), as well as in the residues located near the N terminus of the PHD1 (Tyr294-Val295; Fig. 2c–e ). Similar chemical shift perturbations were observed in the context of H3 peptide binding to the PHD1 of KDM5B (refs 33 , 34 ). Figure 2: Structure and H3 binding properties of KDM5A PHD1. ( a ) Backbone regions of the HSQC spectra of the apo and H3-bound forms of KDM5A PHD1. The apo and H3-bound spectra are coloured blue and orange, respectively. Insets show titration across key structural regions. ( b ) CS-Rosetta model of the apo KDM5A PHD1, consistent with the lowest energy and dihedral restraint considerations. ( c ) Normalized change in chemical shift (Hn, N, Hα, Cα and Cβ) by residue on H3 binding. Dashed lines indicate 25th, 50th and 75th percentile rankings, and colour gradient is such that unperturbed (<25th percentile) positions are in blue and significantly perturbed (>75th percentile) are in orange. ( d ) CS-Rosetta model of KDM5A PHD1 with backbone amides drawn as spheres, coloured by chemical shift perturbation. Selected residue numbers are indicated. ( e ) Surface representation of the KDM5A PHD1 coloured by chemical shift perturbations reveals the H3 binding surface. ( f ) Sequence alignment of KDM5A PHD1 to close homologues. Zinc coordinating residues are highlighted in grey, the conserved tryptophan in blue and aspartate residues proposed to coordinate H3R2 are highlighted in red. The residues that interact with H3K4 are highlighted in light brown. ( g ) Effect of mutations on KDM5A PHD1 recognition of unmodified H3 peptide (NB=no binding, K D >100 μM. Errors ( n ≥3) represent s.e.m.). Full size image By analyzing the chemical shift perturbations of the PHD1 residues on titration of H3 tail peptide, we were able to identify several residues that contribute to recognition of the H3 tail. Similar to other PHD domains that recognize H3, Trp335 (W335), a highly conserved amino acid (aa) involved in recognition of the N-terminal Ala in H3 is essential for peptide binding since a W335A substitution disrupts H3 binding to PHD1 ( Fig. 2c,f,g ) [24] , [34] , [36] , [37] . We further predict that Asp312 and 315 (D312 and D315), residues that recognize the guanidine moiety of R2 in UHRF1, are important for R2 recognition by KDM5A PHD1 domain ( Fig. 2c,f and Supplementary Fig. 7 ) [38] , [39] , [40] , [41] . Consistent with our prediction, mutations D312A and D315A in the PHD1 of KDM5A have a detrimental impact on peptide binding ( Fig. 2g ). The large energetic contribution of R2 to binding is further substantiated by our finding that mutation of this residue in the H3 tail peptide to Ala decreases binding affinity more than 25-fold ( Fig. 1d ). Similar to the role of D312 in R2 recognition, the NMR structure of the PHD1 domain of KDM5B indicates a critical role of the corresponding D328 in forming a salt bridge with R2 of the H3 tail [34] . The substitution of R2 by alanine in this system decreases binding to the H3 tail by ~30-fold ( Fig. 1d ). Structural comparison of unmethylated H3K4 PHD readers Given that the PHD1 domain of KDM5A preferentially recognizes unmethylated H3K4 tail peptide, we compared this domain with other PHD domains that preferentially interact with an unmodified H3K4 tail (for example, PHD1 of KDM5B, BHC80 and AIRE; Fig. 2f ) [24] , [34] , [37] . While recognition of unmodified Lys4 by BHC80 and AIRE PHD domains is achieved by hydrogen bonds with two polar residues and the amino group of Lys4 (D297 side chain and N295 backbone in AIRE and D489 side chain and E488 backbone in BHC80; Fig. 2f and Supplementary Fig. 7 ) [24] , [36] , [37] , [42] , recognition of the Lys4 by the PHD1 domain of KDM5B occurs by a hydrogen bond with Asp308 and two hydrophobic interactions with L325 and Y310 (ref. 34 ). Our NMR studies indicate large chemical shift perturbations of Y294 in the PHD1 of KDM5A (corresponding to Y310 in KDM5B) and the adjacent V295, consistent with their role in direct binding ( Fig. 2c,d,e ). Interestingly, the PHD1 domain of KDM5A can accommodate an alanine at position 4 in the H3 tail peptide with no measurable effect on affinity, as compared with the wild-type (WT) H3 tail peptide ( Fig. 1d ). We speculate that lysine methylation selectivity is achieved mainly by steric occlusion of higher order methylation states at this residue in H3 tail. Together, our CS-Rosetta modelling and chemical shift perturbation studies define the H3 binding pocket of KDM5A PHD1 ( Fig. 2e ) and reveal structural features that explain the large energetic contribution that results from binding of R2. The critical importance of R2 recognition by the PHD1 domains of both KDM5A and KDM5B and their preference for unmodified Lys4 (refs 33 , 34 ) emphasizes potential generality of the function of the PHD1 domains across KDM5 family. KDM5A activty requires a functional PHD1 domain Our biochemical and structural data indicate that mutation of the tryptophan 335 to alanine (W335A) abrogates the binding of the PHD1 to H3K4 tail peptides ( Fig. 2g ). We therefore used this mutation to ask whether the observed stimulation of KDM5A 1–797 -mediated demethylation of the H3K4me3 tail peptides is lost in an enzyme that has a recognition-impaired PHD1 domain. While the W335A mutation does not disrupt the overall fold and stability of either PHD1 or KDM5A 1–797 ( Supplementary Fig. 8 ), consistent with our data, binding of H3 peptides to the W335A mutant of KDM5A 1–797 is abrogated ( Fig. 3a ). More importantly, only the WT KDM5A 1–797 , and not the PHD1-binding-impaired W335A mutant demethylase, is stimulated by the H3 1–18 peptide ( Fig. 3b ). By investigating the demethylation activity of this PHD1 binding-deficient mutant of KDM5A, we found that the catalytic efficiency of KDM5A 1–797 W335A is strongly impaired when compared with the WT enzyme ( Fig. 3c and Supplementary Table 1 ). These experiments indicate that disruption of the PHD1 function in the context of the demethylase negatively impacts catalysis and that peptide binding to a functional PHD1 is coupled to the catalytic activity of KDM5A. 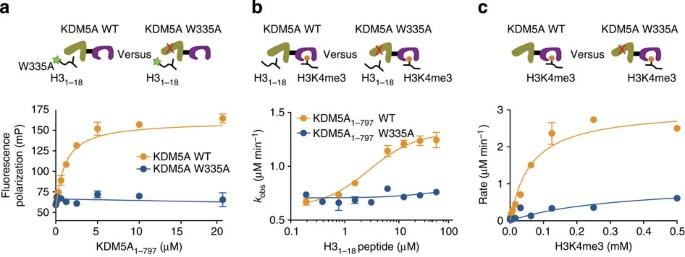Figure 3: Disrupting the function of the PHD1 abrogates the catalytic activity of KDM5A. (a) Binding of WT KDM5A1–797and W335A KDM5A1–797to H3K4me0 tail peptides. (b) Stimulation of H3K4me3 demethylation by WT and W335A KDM5A1–797with increasing concentration of H3K4me0 effector tail peptides. (c) Demethylation activity of WT KDM5A1–797and W335A KDM5A1–797towards H3K4me3 histone tails. Errors (n≥3) represent s.e.m. Figure 3: Disrupting the function of the PHD1 abrogates the catalytic activity of KDM5A. ( a ) Binding of WT KDM5A 1–797 and W335A KDM5A 1–797 to H3K4me0 tail peptides. ( b ) Stimulation of H3K4me3 demethylation by WT and W335A KDM5A 1–797 with increasing concentration of H3K4me0 effector tail peptides. ( c ) Demethylation activity of WT KDM5A 1–797 and W335A KDM5A 1–797 towards H3K4me3 histone tails. Errors ( n ≥3) represent s.e.m. Full size image PHD1 occupancy stimulates nucleosome demethylation Taken together, these experiments demonstrate that peptide binding to the PHD1 domain stimulates the demethylation activity of KDM5A. To get an estimate of the extent of stimulation, we wished to perform demethylation reactions under single turnover conditions. Compared with multiple turnover conditions used to assay peptide demethylation ( Fig. 1e,g ), where both the product generated in each round of demethylation and the excess substrate could occupy the PHD1 domain, using an excess of demethylase and PHD1 ligand peptide over the substrate allows for direct assessment of the impact of PHD1 domain occupancy on catalysis. The demethylation assays were performed with nucleosomes as demethylation substrates under subsaturating single turnover conditions (See Methods and Supplementary Fig. 9 ). We generated homogeneous H3K4 tri-methylated nucleosomes using native chemical ligation between an H3(1–14) thioester peptide tri-methylated on K4 and expressed N-terminally truncated H3(A15C 15–135) protein ( Fig. 4a ). Following desulfurization, the resulting K4 tri-methylated H3 was incorporated into recombinant nucleosomes [43] ( Fig. 4a ). Nucleosome demethylation was assayed by quantitative Western blot-based method that monitors disappearance of the H3K4me3 signal normalized to histone H4, in analogy to a similar assay that we previously developed [44] . It is important to note that, under assay conditions, the antibody was specific for H3K4me3 mark and that no cross-reactivity against H3K4me2 and H3K4me1 modifications was observed ( Supplementary Fig. 10 ). 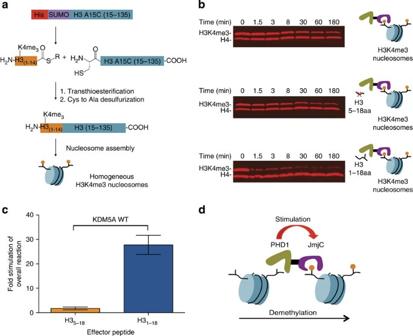Figure 4: Occupancy of the PHD1 by unmodified H3 tail stimulates the demethylation activity of KDM5A on nucleosomes. (a) Preparation of homogeneous H3K4me3 nucleosomes via native chemical ligation and nucleosome reconstitution. R=benzyl. (b) Demethylation activity of KDM5A1–797towards H3K4me3 nucleosomes by quantitative Western blot analysis in the absence or presence of different H3 tail peptides. The conditions used in nucleosome demethylation are as follows: [X]>[E]>[N], [X]>Kdand [N]<Km, where X=H3 tail peptide, E=KDM5A and N=nucleosome;Kdrefers to dissociation constant between the PHD1 domain and the H3 tail peptide andKmto the apparent Michaelis–Menten constant between KDM5A and nucleosomes. (c) Fold stimulation of KDM5A activity on H3K4me3 nucleosome by the addition of different H3 tail peptides. The fold stimulation was obtained by comparing the rate observedkobsin the presence of the effector peptide (H31–18or H35–18) relative to the rate observed in the absence of effector peptide. Errors (n≥3) represent s.e.m. (d) Model for a positive-feedback regulation in KDM5A: newly generated H3K4me0 nucleosomes bind to the PHD1 domain of KDM5A. Occupancy of the PHD1 domain then stimulates the demethylase activity by an allosteric mechanism. Figure 4: Occupancy of the PHD1 by unmodified H3 tail stimulates the demethylation activity of KDM5A on nucleosomes. ( a ) Preparation of homogeneous H3K4me3 nucleosomes via native chemical ligation and nucleosome reconstitution. R=benzyl. ( b ) Demethylation activity of KDM5A 1–797 towards H3K4me3 nucleosomes by quantitative Western blot analysis in the absence or presence of different H3 tail peptides. The conditions used in nucleosome demethylation are as follows: [X]>[E]>[N], [X]> K d and [N]< K m , where X=H3 tail peptide, E=KDM5A and N=nucleosome; K d refers to dissociation constant between the PHD1 domain and the H3 tail peptide and K m to the apparent Michaelis–Menten constant between KDM5A and nucleosomes. ( c ) Fold stimulation of KDM5A activity on H3K4me3 nucleosome by the addition of different H3 tail peptides. The fold stimulation was obtained by comparing the rate observed k obs in the presence of the effector peptide (H3 1–18 or H3 5–18 ) relative to the rate observed in the absence of effector peptide. Errors ( n ≥3) represent s.e.m. ( d ) Model for a positive-feedback regulation in KDM5A: newly generated H3K4me0 nucleosomes bind to the PHD1 domain of KDM5A. Occupancy of the PHD1 domain then stimulates the demethylase activity by an allosteric mechanism. Full size image To test whether occupancy of the PHD1 stimulates KDM5A demethylation activity on nucleosomes, we monitored nucleosome demethylation in the presence of H3 1–18 peptide or truncated H3 5–18 peptide ( Fig. 4b,c ). The addition of H3 1–18 , but not binding-impaired H3 5–18 , stimulates KDM5A demethylation on nucleosomes by ~30-fold ( Fig. 4c ). These results indicate that binding of the unmodified H3 tail to the PHD1 domain stimulates the catalytic activity of KDM5A and further support a model whereby the function of the PHD1 reader domain and the JmjC catalytic domain are energetically coupled ( Fig. 4d ). The presence of both reader and catalytic domains in chromatin-modifying enzymes and/or complexes containing these enzymes has important regulatory implications in chromatin biology. Previous results have demonstrated the role of reader domains in the association of histone demethylases to chromatin. For example, BHC80, a PHD domain-containing protein within the LSD1 co-repressor complex, preferentially binds unmethylated K4 and stabilizes the recruitment of LSD1 to chromatin [24] . Similarly, a double tudor domain of a jumonji histone demethylase KDM4C recruits this demethylase to regions that contain H3K4me3 marks [45] , [46] . In addition, reader domains can regulate substrate specificity of demethylases as in the case of KDM7A and KDM7B (ref. 25 ). Here we show that the function of reader domains in demethylases expands beyond these roles. Using a combination of biochemical and structural studies, we show that the PHD1 domain preferentially recognizes unmethylated H3K4 histone tails, the product of KDM5A-mediated H3K4me3 demethylation. Binding of unmethylated H3K4 peptide by PHD1 stimulates the catalytic activity of KDM5A. This effect is particularly pronounced on homogeneous H3K4me3 nucleosomes as demethylation substrates, where we observe a strong stimulation of KDM5A activity in the presence of PHD1 ligand peptide. We further show that the affinity of the PHD1 domain of KDM5A for histone H3 is modulated not only by methylation of K4 but also by methylation of R2, suggesting an additional layer of regulation of the catalytic activity by the PHD1–H3 tail complex. Our findings are consistent with a model where product recognition by the PHD1 domain allosterically stimulates the catalytic activity of the enzyme on chromatin ( Fig. 4d ). Following initial demethylation events, likely enabled by a combination of the basal activity of the catalytic domain and binding of di- and tri-methylated H3K4 nucleosomes to the PHD1 domain, binding to the resulting H3K4me1/me0 nucleosomes enhances the catalytic activity of KDM5A on the remaining H3K4me3 nucleosomes. Concerted recognition of the product and the substrate by two distinct domains within the same enzyme suggests a model by which demethylation could propagate along nucleosomes through a positive-feedback regulatory mechanism. Positive-feedback regulatory mechanisms have previously been described in several histone methylation complexes and implicated in the propagation of methylation on chromatin. For example, a functional cross-talk between EED, a product-binding WD40 reader subunit of the polycomb repressive complex 2 (PRC2), and the catalytic subunit of the complex, the EZH2 methyltransferase, enables the propagation of H3K27 methylation on chromatin [47] . Similar mechanisms also exist for the Suv39h class of histone methyltransferases, the enzymes that add di- and tri-methyl marks to H3K9 (refs 48 , 49 , 50 ). Our findings that the catalysis of KDM5A is regulated by a positive-feedback mechanism may be particularly relevant in the context of the transcriptional regulation of the HOX gene clusters, known targets of KDM5A-dependent silencing, which contain large Lys 4 methylated regions [13] , [51] , [52] , [53] . An alternative, but not mutually exclusive, possibility is that occupancy of the PHD1 domain by the histone tail may stabilize the composite active site formed by JmjN and JmjC domains and, in doing so, contribute to enhance the basal activity of the demethylase. While various modified H3 tails could serve as ligands, optimal stimulation is only achieved by an unmethylated H3K4 tail, given that in its unmodified state the H3 tail has the highest affinity for the PHD1 ( Fig. 1c,d,f ). Given the high sequence homology of the PHD1 reader domains across members of KDM5 family [30] , [33] , we hypothesize that the functional role of the PHD1 in regulating KDM5A catalysis is conserved among KDM5 enzymes. If conserved, our findings can help explain previous in vivo observations that the deletion of the PHD1 in the Drosophila KDM5 homologue Lid abrogates its catalytic activity in cells [29] , [30] . In addition, it was recently shown that abrogation of H3 tail recognition by point mutation in the PHD1 domain of KDM5B decreases H3K4 demethylation in cells, resulting in the repression of tumour suppressor genes by approximately twofold [34] . We anticipate that future mechanistic and structural studies aimed at understanding the functional cross-talk between catalytic and ligand binding domains in KDM5 enzymes will help to better elucidate the role of this cross-talk in the regulation of H3K4 methylation in a cellular context. Finally, given the oncogenic function of KDM5A in several cancers and its role in drug resistance in cancer, the identification of an allosteric regulatory site provides an attractive opportunity for the development of small molecule allosteric modulators of the activity of this enzyme. Expression of recombinant H3 C-terminal fragment SMT3(1–98) followed by C-terminal H3 fragment H3 (15–136 A15C) was cloned into pET28b (NheI-BahmHI) and transformed in Rosetta (DE3) pLysS. Cells were grown at 37 °C to an OD 600 of ~0.6 and induced with a final concentration of 0.4 mM isopropyl β-D-1-thiogalactopyranoside for 3 h. Cells were harvested and lysed by sonication. Pelleted inclusion bodies were washed twice with wash buffer (50 mM Hepes pH 7.5, 100 mM NaCl, 1 mM EDTA and 1 mM benzamidine) containing 1% Triton X-100 and twice with wash buffer without detergent. Inclusion bodies were extracted with unfolding buffer (7 M guanidinium HCl, 20 mM Hepes pH 7.5 and 10 mM dithiothreitol (DTT)) and incubated with Ni:NTA. The resin was washed with 10 column volumes of high salt buffer (2 M urea, 20 mM sodium acetate pH 5.2, 1 M NaCl, 5 mM β-mercaptoethanol (βME) and 25 mM imidazole) and 2 column volumes of cleavage/dilution Buffer (2 M Urea, 2 mM DTT, 150 mM L-Arg, 10 mM L-Cys, 150 mM NaCl and 50 mM Hepes pH 6.8). Protein was eluted in cleavage/dilution Buffer containing 250 mM imidazole. Eluted protein was diluted so that the final concentration was ~0.25 mg ml −1 and imidazole concentration was <150 mM. Approximately 1:10 of Senp-SUMO(419–644) protease to protein was added while dialyzing in water containing 5 mM BME. Cleaved C-terminal H3 fragment was lyophilyzed and further purified by semi preparative C-18 RP-HPLC using a 0–60% acetonitrile (ACN) with a 0.1% trifluoroacetic acid gradient for 1 h. Native chemical ligation and desulfurization of H3K4me3 Native chemical ligation was performed essentially as previously described [54] . Briefly, 11.1 mg (0.804 μM, 1 equiv.) of H3 (aa 15–136 A15C) was dissolved in 518 μl of ligation/desulphurization buffer (200 mM sodium phosphate pH 7.8, 6 M guanidinium HCl). Dissolved histone was reduced with 28 μl of 1 M Tris(2-carboxyethyl)phosphine TCEP (~50 mM) for 1 h at 37 °C. Then 9.25 mg (~100 mM) of 4-mercaptophenylacetic acid (MPAA) and (2.2 μmol, 2.8 equiv.) of H3K4me3-(S-benzyl) 14-mer (AnaSpec Inc.) were added, flushed with Argon and left to react while vigorously stirring at 50 °C until the completion of the reaction (typically overnight). The product was purified by semi preparative C-18 RP-HPLC using a 0–60% ACN with a 0.1% TFA gradient for 1 h. Desulfurization of cysteine 15 to the native alanine was performed by a free-radical-based approach [54] , [55] . In a typical reaction, 1 mg of H3K4me3 A15C was dissolved in 114 μl of the ligation/desulphurization buffer (200 mM sodium phosphate pH 7.8, 6 M guanidinium HCl). About 20 μl of 400 mM reduced glutathione, 50 μl of 1 M TCEP and 6 μl of 0.2 M VA-061 (Wako Chemicals) radical initiator in methanol were added. Reaction mixture was flushed with Argon and left to react at 37 °C overnight. The product was purified by semi preparative C-18 RP-HPLC using a 0–60% ACN with a 0.1% TFA gradient for 1 h. Nucleosomes assembly Except for H3K4me3, full length histones H2A, H2B and H4 were recombinantly expressed and purified under denaturing conditions [43] . H3K4me3 nucleosomes were assembled on 147 bp of DNA using the 601 positioning sequence. The DNA was amplified by PCR and gel purified. The DNA fragment was assembled into mononucleosomes with recombinant Xenopus laevis histones by salt dialysis [43] . Expression of recombinant GST–PHD1 (aa 291–347) GST-tagged PHD1 (aa 291–347) protein was expressed in E. coli BL21-Gold (DE3) in 2 × YT broth (2 × Yeast extract and Tryptone) via isopropyl β-D-1-thiogalactopyranoside induction overnight at 18 °C. Cells were resuspended in 140 mM NaCl, 2.7 mM KCl, 10 mM Na 2 HPO 4 , 1.8 mM KH 2 PO 4 , 5 mM βME, 50 μM ZnCl2, 1 mM Phenylmethylsulfonyl fluoride PMSF pH 7.3, lysed by sonication and centrifuged. The supernatant was purified using a Glutathione Separose 4B resin, washed with high salt buffer (50 mM Hepes pH 8, 700 mM KCl, 10% glycerol, 5 mM βME, 50 μM ZnCl 2 , 1 mM PMSF) and low salt buffer (50 mM Hepes, 150 mM KCl, 10% glycerol, 5 mM βME, 50 μM ZnCl 2 , 1 mM PMSF pH 8) and recovered by elution using low salt buffer with 30 mM glutathione. The sample was dialyzed overnight in 40 mM Hepes, 50 mM KCl, 0.5 mM TCEP and 50 μM ZnCl 2 . Protein was further purified by anion exchange on MonoQ 10/100 with a linear gradient of low salt buffer (40 mM Hepes, 50 mM KCl, 0.5 mM TCEP and 50 μM ZnCl 2 ) and high salt buffer (40 mM Hepes, 1 M KCl, 0.5 mM TCEP and 50 μM ZnCl 2 ). Thermal shift assay The thermal denaturation of WT and mutant proteins was monitored indirectly by a fluorescence-based thermal shift assay using SYPRO orange dye in a buffer containing 50 μl of 1 μM protein with 1/5,000 SYPRO orange in 50 mM Hepes, 50 mM KCl pH 7.5. The plate was heated from 25 to 95 °C with a heating rate of 1 °C/min. The fluorescence intensity was measured with exication/emission of 492/590 nm, respectively. Far-ultraviolet circular dichroism spectrophotometry Far-ultraviolet circular dichroism measurements were recorded on a Jasco J-715 spectropolarimeter at 11 °C using 1-mm path length from 300 to 200 nm with a scan speed of 50 nm min −1 , three scans and 3 ml, 320 nM for GST-PHD1 WT and W335A or 145 nM for KDM5A 1–797 WT, W335A in buffer (20 mM KH 2 PO 4 pH 7.5 10 μM Fe(NH 4 ) 2 (SO 4 ) 2 , 100 mM ascorbate). The spectra were corrected for buffer. FP studies The association of GST-PHD1 291–347 with H3 1–18 was measured by either direct or competition-based FP. All measurements were obtained in a buffer containing 50 mM Hepes pH 7.5, 50 mM KCl and 0.01% Tween-20 at 25 °C. The binding mixture was incubated for 30 min at room temperature and FP was measured using a Molecular Devices HT Analyst with excitation and emission wavelengths of λ ex 480 nm and λ em 530 nm, respectively. All data were visualized using Graphpad Prism. For direct FP binding assay, 10 nM of C-terminal fluorescently labelled H3 peptide (GenScript) were incubated with varying concentrations of GST-PHD1 291–347 . Data were analyzed as previously reported in Canzio et al. [56] For competition-based FP assays, 2 μM GST-PHD1 291–347 was incubated with 10 nM of C-terminal fluorescently labelled H3 peptide and different concentrations of unlabelled peptides were used as competitors. All data were visualized using Graphpad Prism and analyzed using the following model adapted from Narlikar et al. [57] : Baculoviral expression and purification of KDM5A 1–797 KDM5A (aa 1–797) was expressed in sf21 cells following Invitrogen Bac-to-Bac Baculovirus expression system protocol. KDM5A 1–797 was cloned into a pFASTBAC HTA vector following a ligation-independent PCR cloning method [58] . Purified bacmid was transfected in sf21 cells. Approximately 0.8 × 10 −5 cells per well of a six-well dish were allowed to attach in 2 ml of SF-900 II SFM media containing 50 U ml −1 penicillin and 50 μg ml −1 streptomycin. While cells attached, 8 μl of Cellfectin II reagent (Invitrogen) in 100 μl of unsupplemented Grace’s Medium was mixed with ~2–5 μg of bacmid in 100 μl of unsupplemented Grace’s Medium and incubated for 15–30 min at 25 °C. Once cells were attached, media was removed and cells were washed with 2 ml of Grace’s unsupplemented media. The Bacmid DNA:Cellfectin mixture was then diluted to 1 ml with Grace’s unsupplemented media and added to the well. Cells with Bacmid:Cellfectin II mixture were incubated for 5 h at 27 °C. After 5 h of incubation, bacmid:Cellfectin mixture was removed and replaced with 2 ml of SF-900 II SFM 50 U ml −1 penicillin and 50 μg ml −1 streptomycin. Transfected cells were incubated 3–5 days or until signs of viral infection were observed. After transfection, the supernatant was spun down to remove the dead cells. The supernatant was then sterile filtered to obtain the P1 viral stock. To make P2, 20 ml of viral stock at ~2 × 10 6 cells per ml of sf21 was infected with 2 ml of P1 virus and incubated for 48–60 h. After 56 h, the cells were spun down and the supernanant was collected and sterile filtered to obtain P2 viral stock. Similarly, P3 viral stock from P2 viral stock was obtained. Generally, 1 l of sf21 at 2 × 10 6 cells per ml was infected with ~40 ml of P3 virus for ~48–56 h. Cells were then collected and resuspended in the lysis buffer (25 mM Hepes pH 7.9, 350 mM NaCl, 5 mM KCl, 1.5 mM MgCl 2 , 10 mM imidazole, aprotinin 2 μg ml −1 , leupeptin 3 μg ml −1 , pepstatin 3 μg ml −1 , 1 mM PMSF). Cells were homogenized by emulsiflex. After lysis, the supernatant was recovered by centrifuging at 35k r.p.m. for 45 min, and incubated with cobalt resin equilibrated in lysis buffer for 1 h at 4 °C. After incubation the resin was washed with wash buffer (25 mM Hepes, pH 7.9, 350 mM NaCl, 0.5 mM MgCl 2 , 10% glycerol, 10 mM imidazole, aprotinin 2 μg ml −1 , leupeptin 3 μg ml −1 , pepstatin 3 μg ml −1 and 1 mM PMSF). His-KDM5A was eluted with elution buffer (25 mM Hepes pH 7.9, 100 mM NaCl, 0.5 mM MgCl 2 , 10% glycerol, 100 mM imidazole, aprotinin 2 μg ml −1 , leupeptin 3 μg ml −1 , pepstatin 3 μg ml −1 and 1 mM PMSF). The his-tag was removed by overnight incubation with TEV protease at 4 °C in the dialysis buffer (25 mM Hepes, pH 7.9,100 mM NaCl and 2 mM DTT). After cleavage, protein was further purified by size-exclusion chromatography using S200 column. Purified KDM5A was eluted, aliquoted and stored at −80 °C in 40 mM Hepes, pH 7.9, 50 mM KCl. The percentage of Cobalt in purified KDM5A was 24.3%, as determined by inductively coupled plasma mass spectrometric analysis (ActLabs, Ancaster, Ontario). Prior to an experiment, KDM5A aliquots were defrosted in ice and immediately used. Demethylation assay on H3 peptides Demethylation reactions on H3 peptides were performed in a demethylation buffer containing 50 mM Hepes pH 7.5, 50 mM KCl, 1 mM α-ketoglutarate, 50 μM Fe(NH 4 ) 2 (SO 4 ) 2 and 2 mM ascorbic acid. Reactions were performed at room temperature. For the enzyme-coupled assay: 2 mM NAD + and 0.05 FDH (Sigma) were added to the reaction to monitor lysine 4 demethylation of histone H3 by following the production of formaldehyde [35] . Different concentrations of H3K4me3/2/1 peptides (aa 1–18, GenScript) were incubated with 1 μM KDM5A. Reactions were initiated by the addition of substrate and followed in 20-s intervals on a SpectraMax M5e (Molecular Devices) using 350 nm excitation and 460 nm emission wavelengths. An NADH standard curve was used to convert fluorescence to concentration of product formed. The initial 2 min were used to calculate initial velocities, which were plotted against substrate concentration. Michaelis–Menten parameters were determined using Graphpad Prism. For the stimulation assay, the H3K4me3 substrate was kept constant (10 μM) while the concentration of the effector H3 peptides (aa 1–18 or 5–18) was varied. For the mass-spectrometry demethylation assay, 5 μM KDM5A was incubated with 200 μM H3K4me3/2/1 in demethylation buffer. After incubation at room temperature for 3 h, the reaction was quenched by EDTA (final concentration of 5 mM) and incubation at 100 °C for 3 min. Reactions were desalted through C-18 ZipTips (Millipore). The eluted peptide was further diluted ten times in 0.1% formic acid. The extent of demethylation was analyzed by matrix-assisted laser desorption/ionization–time of flight mass-spectrometry using 2,5-dihydroxybenzoic acid as matrix. Subsaturating single turnover nucleosome demethylation assay Demethylation reactions on nucleosomes were carried out using 300 nM H3K4me3 nucleosomes and 3 μM KDM5A in the presence or absence of 12.5 μM H3 1–18 or H3 5–18 in the demethylation buffer (50 mM Hepes pH 7.5, 50 mM KCl, 1 mM α-ketoglutarate, 50 μM Fe(NH 4 ) 2 (SO 4 ) 2 and 2 mM ascorbic acid). The experiment was performed under subsaturating single turnover conditions where the effector peptide (H3 1–18 ) is above its K d to the PHD1 domain and KDM5A is 10-fold above H3K4me3 nucleosome concentration. Reactions were initiated by the addition of methylated nucleosomes and quenched with 6 × SDS sample loading buffer and 0.5 M EDTA, pH 8.0. The reaction mixture was analyzed by Western blotting using anti-H3K4me3 (1:2,000, Millipore cat# 05–1339) anti-H4 (1:1,400, Abcam cat# ab31830), IRDye 680 LT goat polyclonal anti-mouse immunoglobulin-G (1:20,000, Licor cat# 926–68020). All data were visualized using Graphpad Prism and analyzed as previously reported in Shiau. et al. [44] Nuclear magnetic resonance A minimal PHD1 construct of KDM5A (D292—E344) was used in the structural studies. This 6 × -His-TEV-PHD1 was expressed in M9 minimal media containing 15 N ammonium chloride and 13 C 6 -D-glucose. The 13 C-/ 15 N-enriched protein was purified as described for the binding studies with the additional steps of TEV protease cleavage and anion exchange chromatography via HiTrap Q (GE Healthcare). 3D triple-resonance experiments for backbone assignment (HNCACB (pulse programme: hncacbgpwg3d, TopSpin1.3p18) and CBCA(CO)NH) (pulse programme: cbcaconhgpwg3d, TopSpin1.3p18) [59] and 3D quantitative-J HNHA (pulse programme: hnhagp3d, TopSpin 1.3p18) [60] experiments were recorded with a 500 MHz Bruker AVANCE DRX500 spectrometer equipped with a Z-gradient QCI cryoprobe ( 15 N/ 13 C/ 31 P, 1 H). The 2D [ 15 N, 1 H]-HSQC (pulse programme: fhsqcf3gpph, TopSpin1.3p18) [61] spectra for the H3K4me0(1–10) titration series were recorded on an 800 MHz Bruker AVANCEI spectrometer equipped with a Z-gradient TXI cryoprobe. The 3D spectra were processed in NMRPipe [62] and proton chemical shifts were referenced to a DSS standard and 13 C and 15 N were referenced indirectly to this value [63] . Resonance assignments and data analysis, including prediction of ψ and ϕ dihedral angles from chemical shifts using DANGLE [64] and extraction of 3 J-HNHA ( ϕ ) coupling constants, were performed with CCPNMR [65] . The 3D experiments for the assignment of Apo PHD1 used a 180 μM PHD1 sample; 2D 15 N-HSQC titration spectra were collected with a 55 μM PHD1 sample ([H3K4me0] ranged from 11 to 260 μM) and the experiments for the assignment of H3-bound PHD1 were acquired with a 160 μM PHD1 sample containing 2 mM H3K4me0. Assignment of the H3-bound PHD was deemed critical for correct mapping of peaks that broadened (underwent intermediate time scale exchange) during the titration points prior to saturation. See Supplementary Fig. 6 for high resolution HSQC spectra of all titration points. In calculation of per residue chemical shift perturbation, all recorded chemical shifts were considered and normalized with the following equation: All experiments were carried out at 298 K (calibrated with 4% v/v MeOH in MeOD) in 50 mM Hepes, 150 mM NaCl, 0.5 mM TCEP and 0.1 mM ZnCl 2 at pH 7.5 in 5% D 2 O. Chemical shifts for the apo and H3-bound KDM5A PHD1 will be deposited in the Biological Magnetic Resonance Data Bank. CS-Rosetta model calculations After assignment in CCPNMR, chemical shifts for 1 H, 15 N, 1 Hα, 13 Cα and 13 Cβ of the apo PHD1 protein were submitted to the BMRB CS-Rosetta web server for generation of fragment libraries. The chemical shift-selected fragments were then used in Rosetta ab initio structure prediction (Rosetta v3.5). Simulations included restraints for the metal coordination of the two Zn-binding sites [66] , and stereochemistry of the chiral zinc centres was inferred by comparison with homologous structures. For the apo structure predictions, 30,975 starting decoys were generated with the ab initio protocol. These decoys were ranked by energy and the top 5,000 were further optimized using a fast relax protocol, generating an additional 25,000 decoys. These models were then filtered by score using the all-atom Rosetta force field, and only the lowest scoring fast relax models from the 5,000 ab initio models were included with the ab initio set. Rosetta decoys were sorted by score and all residue pairwise Cα RMSDs were calculated for this set of 35,975 Rosetta decoys using fast_protein_cluster [67] . For a flow chart of CS-Rosetta model generation see Supplementary Fig. 3a . Plotting the Rosetta all-atom energy as a function of RMSD (to the lowest energy model) did not reveal the drop in energy at low RMSD values (‘funnel’ shape) typically observed for well-converged simulations, when Cα RMSDs were computed over the entire length of the PHD domain ( Supplementary Fig. 3b ). However, recalculation of Cα RMSD using different regions of the domain produced the characteristic funnel shape that is typical for successful structural prediction [68] . The converged regions are those of well-defined secondary structure (the core beta-sheet and the C-terminal alpha-helix; Supplementary Fig. 4 ). The top 50 models by Rosetta all-atom energy were compared with the measured dihedral restraints ( 3 J HN-HA ; Supplementary Table 2 ), and only those with violations <15° were included in the structural ensemble ( n =8) used in the comparison with other known PHD finger structures. Comparison to structurally determined homologous PHD fingers In superposition of the KDM5A ensemble of decoys and all closely related PDB homologues, the structural core of the domain is well-conserved. However, the extended/‘open’ conformation of the L2 loop appears unique to KDM5A ( Supplementary Fig. 5 ). The L2 loop was defined as spanning residues 322 through 337. The centres of mass for these regions were calculated by taking the mean Cα position of residues within these regions across each individual model. The relative position of the L2 loop was determined by calculating the center of mass of the zinc ligands ( Supplementary Fig. 5a-c ). This angle ( θ ) then defines the relative position of the L2 loop with respect to the core of the PHD finger, with small theta presenting as a compact/‘closed’ form and large theta giving a more extended/‘open’ form. The angle theta was calculated for the CS-Rosetta ensemble and the homologous structures and these distributions are presented in Supplementary Fig. 5d . How to cite this article: Torres, I.O. et al. Histone demethylase KDM5A is regulated by its reader domain through a positive-feedback mechanism. Nat. Commun. 6:6204 doi: 10.1038/ncomms7204 (2015).